Synthesis of chiral TiO2nanofibre with electron transition-based optical activity The optical chirality induced at the absorption bands due to electronic exciton coupling of the transition dipole moments between chromophores in close proximity is ubiquitous in helical organic materials. However, inorganic materials with optical activity resulting from electronic transitions have not been explored. Here we report the synthesis of chiral TiO 2 fibres via transcription of the helical structure of amino acid-derived amphiphile fibres through coordination bonding interactions between the organics and the TiO 2 source. Upon calcination, the as-prepared amorphous TiO 2 double-helical fibres with a pitch length of ~100 nm were converted to double-helical crystalline fibres with stacks of anatase nanocrystals in an epitaxial helical relationship. Both the amorphous and anatase crystalline helical TiO 2 fibres exhibited optical response to circularly polarized light at the absorption edge around ~350 nm. This was attributed to the semiconductor TiO 2 -based electronic transitions from the valence band to the conduction band under an asymmetric electric field. The optical activity (OA) of materials arises from the ability of a medium to have different interaction for left and right circularized light [1] , [2] , [3] , [4] , [5] , [6] . Various chiral inorganic materials with scattering-, refraction- and absorption-based OA have been investigated extensively. Scattering at the inorganic/air interfaces of the helical arrays, such as for chiral films of MgF 2 , TiO 2 and SiO 2 , tends to transmit circularly polarized light of one handedness and reflect the other in a wavelength, which depends on the pitch length and effective refractive index [1] , [2] , [7] , [8] , [9] ; while refraction by the helical arrangement of the basic building blocks, such as chiral crystals of quartz, NaClO 3 and NaBrO 3 , results in different velocities of right- and left-handed circularly polarized light in the medium [3] . These scattering-based OA and refraction-based OA are related to the geometry and refractive index regardless of the type of inorganics. For the absorption-based OA inorganic materials, although inorganic nanoparticles functionalized with chiral organic molecules and assembled helically in organic assemblies gave rise to OA in their visible absorption region, such OA is due to plasmon oscillations of the excited electron in the given metal nanoparticles, and disappeared after removing the organics [10] , [11] , [12] . Therefore, it is still a challenge to explore new types of optically active inorganic materials featuring optical, electrical, mechanical and biological properties. As known, molecular electronic transitions in organic and inorganic compounds occur when electrons are excited from a lower energy level to a higher energy level, which results in absorption of the electromagnetic wave with the corresponding energy difference between the two levels covering a wide energy range. In organic materials that have a helical geometry, the electronic transition-based optical activity (ETOA) at the absorption bands due to electronic exciton coupling is ubiquitous. However, although many inorganic materials exhibit electronic transitions in the ultraviolet or visible range of the electromagnetic spectrum, no electronic transition-based optically active inorganic materials have been reported up to now. Several macroscopic helical morphologies of inorganic materials were successfully synthesized by templating methods to transcribe organic molecules or assemblies onto inorganic materials (for example, semiconductors [13] , [14] , metal oxides [15] , carbonates [16] and mesoporous silica materials [2] , [17] , [18] ), which might have molecular chirality with OA similar to organics. However, in contrast to organic materials, all of these materials do not result in OA at the absorption bands, probably because either non-photosensitive inorganics have been used or large pitch length has been formed. In this investigation, TiO 2 was used to study the ETOA of inorganic materials, as the anatase form typically exhibits ultraviolet absorption in the region of 200–400 nm. We synthesized chiral TiO 2 with a pitch length shorter than 100 nm via a templating method to transcribe the helical structure of lipid fibres onto the microscopic helical assembly of inorganic TiO 2 . Lipid amphiphilic molecules of N -acylamino acids with hydrophobic chains were used as a template, which can self-organize to form helical ribbons or fibres with a bilayer molecular arrangement [19] . In particular, titanium diisopropoxide bis(acetylacetonate) (TDA) was used as the TiO 2 source to achieve full interaction between template and inorganic species for effective transcription by decreasing condensation rate. In our previous work, the helical lipid aggregation of N -acyl- L -glutamic acid (C n - L -Glu) was shown to template chiral mesoporous poly(pyrrole) with a short pitch length of 100 nm through fine electrostatic interactions between the negatively charged head groups of the lipid amphiphilic molecules and the positively charged imine nitrogens of poly(pyrrole) [19] . Decreasing the repulsion between the negatively charged carboxylate head groups to allow closer interactions was the key to the formation of a short pitch length. The strategy used in this investigation to synthesize chiral TiO 2 with a short pitch length was to control the interaction between the carboxylic head groups of C n - L / D -Glu and the TiO 2 species. Conventional TiO 2 sources are generally considered to be inappropriate for the synthesis of TiO 2 fibres because the hydrolysis rates of these titanium salts and alkoxides, as well as the condensation rates of the highly reactive M–OH species, are too rapid. The high rates lead to continuous/homogeneous nucleation and growth, and the TiO 2 never interacts with other ligands. Thus, organic templating is extremely difficult. If a slow, controlled nucleation can be driven and fine interactions with carboxylic acids maintained, then TiO 2 fibres can be templated by carboxylic acid amphiphilic molecules. The coordination bonding would allow closer interactions between carboxylate head groups similar to the formation of mesoporous poly(pyrrole), and thus resulted in short pitch length [19] . The hydrolysis of TDA occurs slowly in the pH range of 3–8. The synthetic system used in this report relied upon the use of TDA to decrease the rate of the hydrolysis and condensation reactions of the TiO 2 source. Additionally, interactions between lipid helical fibres through the titanium–carboxylic acid (Ti-COOH) coordination at the interface would result in the formation of lipid–TiO 2 hybrid helical fibres. Through calcination, the organic lipid can be subsequently removed, and the amorphous TiO 2 can be transformed to a pure inorganic crystalline phase. Here, the synthesis of chiral TiO 2 fibres was achieved via transcription of the helical structure of amino acid-derived amphiphile fibres through fine coordination bonding interactions between the carboxylic groups and the TiO 2 source. The amorphous and crystal TiO 2 double-helical fibres exhibited optical response to circularly polarized light at their absorption bands, which was attributed to the semiconductor TiO 2 -based electronic transitions from the valence band to the conduction band under an asymmetric electric field. Structure of chiral lipid–TiO 2 hybrid nanofibres Antipodal lipid–TiO 2 hybrids with a pale yellow colour were synthesized using N -stearoyl- L / D -glutamic acid (C 18 - L / D -Glu) lipid enantiomers as the template and TDA as the TiO 2 source in a methanol/water solution (see the Methods section). As shown in Fig. 1a and b , scanning electron microscopy (SEM) revealed that the as-prepared lipid–TiO 2 hybrid that was synthesized with C 18 - D -Glu was exclusively composed of right-handed double-helical fibres. The width of a single fibre was ~25 nm. From the distinct helical morphology, the pitch along the axis of the fibre was estimated to be ~100 nm, which is indicated by the distance between the two black (or white) arrows. The C 18 - L -Glu molecule gave mirror-image profiles with the same size and quality ( Supplementary Fig. 1 ). The as-prepared left- and right-handed lipid–TiO 2 hybrid fibres are denoted as L-TiO 2 -as and R-TiO 2 -as, respectively. 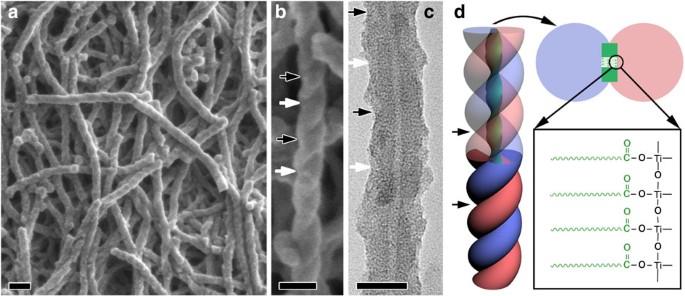Figure 1: Microscopy and schematic drawings of the as-prepared organic lipid–TiO2hybrid fibres. SEM images, TEM images and schematic drawings of the as-prepared organic lipid–TiO2hybrid fibres synthesized with C18-D-Glu (R-TiO2-as). The molar composition for the synthesis was C18-D-Glu:TDA:MeOH:H2O=1:7.5:5351:55962. (a,b) SEM images with different magnifications that show the right-handed double-helical microscopic features of the fibres with a pitch length of ~100 nm, as indicated by the distance between the two black (or white) arrow heads (JEOL JSM-7401F). The samples were observed without any metal coating. (c) TEM image that shows a tube in the centre of the fibre. Images were acquired using a JEOL JEM-2100 TEM at 200 kV. (d) Schematic drawing of a structural model of the chiral TiO2tubular fibre, which shows the lamellar structure of the C18-D-Glu rectangular lipid fibre template for the formation of the lipid–TiO2hybrid through fine coordination interaction between the carboxylic acid and titanium. The scale bars ina,bandcrepresent 100, 50 and 10 nm, respectively. Figure 1: Microscopy and schematic drawings of the as-prepared organic lipid–TiO 2 hybrid fibres. SEM images, TEM images and schematic drawings of the as-prepared organic lipid–TiO 2 hybrid fibres synthesized with C 18 - D -Glu (R-TiO 2 -as). The molar composition for the synthesis was C 18 - D -Glu:TDA:MeOH:H 2 O=1:7.5:5351:55962. ( a , b ) SEM images with different magnifications that show the right-handed double-helical microscopic features of the fibres with a pitch length of ~100 nm, as indicated by the distance between the two black (or white) arrow heads (JEOL JSM-7401F). The samples were observed without any metal coating. ( c ) TEM image that shows a tube in the centre of the fibre. Images were acquired using a JEOL JEM-2100 TEM at 200 kV. ( d ) Schematic drawing of a structural model of the chiral TiO 2 tubular fibre, which shows the lamellar structure of the C 18 - D -Glu rectangular lipid fibre template for the formation of the lipid–TiO 2 hybrid through fine coordination interaction between the carboxylic acid and titanium. The scale bars in a , b and c represent 100, 50 and 10 nm, respectively. Full size image High-resolution transmission electron microscopy (HRTEM) image ( Fig. 1c ) indicated that the fibres possess inner tubes with a diameter of ~12 nm that are constant along the central axis of each individual tube. All of the helical tubes were open-ended. The N 2 adsorption–desorption results showed that no pores corresponding to the size observed in the transmission electron microscopy (TEM) image existed in the lipid–TiO 2 hybrid, which indicated that the inner tubes were filled with the lipid ( Supplementary Fig. 2 ). Similar to the chiral mesoporous poly(pyrrole) reported in our previous work [19] , the helical tube was probably the self-assembled, lamellar-structured C 18 - D -Glu rectangular lipid used to template the helical TiO 2 . At first, the carboxylic acid group of the C 18 - D -Glu interacted with the titanium through coordination bonding, and the TiO 2 began templating the helical ribbon, which subsequently induced the formation of a TiO 2 wall. The preferential interaction with both large sides of the rectangular tape led to the formation of double-helical TiO 2 , as shown in Fig. 1d . The presence of coordination bonding was confirmed by Fourier transform infrared spectroscopy ( Supplementary Fig. 3 ). Structure of calcined chiral TiO 2 nanofibres The as-prepared amorphous lipid–TiO 2 hybrids were converted to white crystalline TiO 2 by calcination in air at elevated temperatures. The X-ray diffraction patterns ( Fig. 2 ) showed that the as-prepared fibres were amorphous in structure with essentially no diffraction peaks. However, the TiO 2 obtained after calcination at 550 °C was assigned to the anatase phase (JCPDS File No. 21-1272) without any indication of other crystalline by-products. As can be observed in the SEM image ( Fig. 3a ) of the calcined sample, although the fibres no longer had a smooth surface, the right-handed double-helical morphology remained. The fibres were composed of stacked TiO 2 nanoparticles with an average diameter of ~20 nm, which indicates that an obvious shrinkage occurred during calcination without destruction of the helical structure. The calcined left- and right-handed TiO 2 fibres are denoted as L-TiO 2 -cal and R-TiO 2 -cal, respectively. 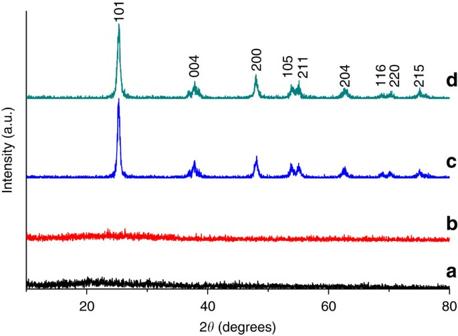Figure 2: X-ray diffraction patterns of as-prepared and calcined chiral TiO2fibres. X-ray diffraction patterns of as-prepared ((a) L-TiO2-as and (b) R-TiO2-as) and calcined ((c) L-TiO2-cal and (d) R-TiO2-cal) chiral TiO2fibres, which indicate that the as-prepared samples were amorphous. The TiO2obtained after calcination at 550 °C was assigned as the anatase phase, and there was no indication of other crystalline by-products. Figure 2: X-ray diffraction patterns of as-prepared and calcined chiral TiO 2 fibres. X-ray diffraction patterns of as-prepared (( a ) L-TiO 2 -as and ( b ) R-TiO 2 -as) and calcined (( c ) L-TiO 2 -cal and ( d ) R-TiO 2 -cal) chiral TiO 2 fibres, which indicate that the as-prepared samples were amorphous. The TiO 2 obtained after calcination at 550 °C was assigned as the anatase phase, and there was no indication of other crystalline by-products. 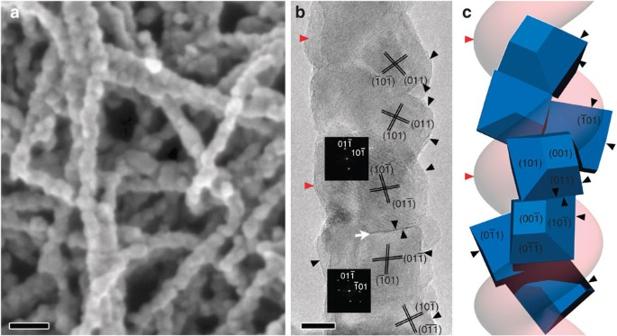Figure 3: Electron microscopy and schematic drawing of calcined chiral crystalline TiO2. (a) SEM image that shows the right-handed helical microscopic features of the sample (JEOL JSM-7401F). (b) The HRTEM image and the corresponding Fourier diffractograms of two nanocrystals. (c) Structural model showing the helical stacking of TiO2anatase nanocrystals and good correspondence with the double-helical morphology. The common facets of the nanocrystals are (011), (101), (101), (011), (101), (011) from top to bottom, respectively. The other strand of the double-helix fibre (pink) is shown without crystal particles. The scale bars inaandbrepresent 50 and 10 nm, respectively. Full size image Figure 3: Electron microscopy and schematic drawing of calcined chiral crystalline TiO 2 . ( a ) SEM image that shows the right-handed helical microscopic features of the sample (JEOL JSM-7401F). ( b ) The HRTEM image and the corresponding Fourier diffractograms of two nanocrystals. ( c ) Structural model showing the helical stacking of TiO 2 anatase nanocrystals and good correspondence with the double-helical morphology. The common facets of the nanocrystals are (011), (101), (101), (011), (101), (011) from top to bottom, respectively. The other strand of the double-helix fibre (pink) is shown without crystal particles. The scale bars in a and b represent 50 and 10 nm, respectively. Full size image The HRTEM image shown in Fig. 3b revealed that the calcined TiO 2 fibres were composed of stacks of small anatase single crystals with an average size of ~20 nm along the long axis of the fibre. It is worthy to note that the SEM image and the adsorption contrast of the TEM image indicate that the calcined fibres generally retained the double-helical morphology of the as-prepared samples. However, the former hollow tubular structures disappeared upon the growth of the anatase nanocrystals. Interestingly, the HRTEM image shows that an array of nanocrystals exhibits the contrast close to ‹111› zone axis of the anatase structure, which indicates that the nanocrystals must have a preferential growth direction during the crystallization process. Besides, a twin boundary, formed by two anatase nanocrystals sharing their common (011) facets, can be clearly observed, as indicated by the white arrow heads. Additionally, it has been observed that the {101} facets of the nanocrystals were often exposed, as indicated by the black arrows in the image. The morphology of anatase crystals are in good agreement with early experimental observations and theoretical calculations, in which the morphologies were dominated by the thermodynamically stable {101} facets (constitutes more than 94% of the crystal surface according to the Wulff construction) and {001} facets [20] . In conclusion, the nanocrystals are formed according to the initially formed double-helical structure and the crystallization to anatase. The double-helical morphology caused the nanocrystals to maintain a chiral packing relationship. Therefore, a possible structural model is established, as shown in Fig. 3c . In particular, the adjacent nanocrystals have a rotational misplaced arrangement, piling up by sharing one of their {101} facets while keeping one of the ‹111› axis in common, leading to a helical array of nanocrystals with almost parallel ‹111› axes. Both the lattice planes and the morphologies of the nanocrystals fit the HRTEM image perfectly (marked by the black arrow heads). However, the contrast-overlap problem observed in the HRTEM image and the small crystal size caused the determination of the structural relationship of all the nanocrystals to be extremely difficult. Even so, it can be deduced that both helical strands have the similar epitaxial relationship and the TiO 2 fibres generally still possess the double-helix chiral packing feature. Further investigation is still under way. OA of chiral lipid–TiO 2 hybrid and pure TiO 2 nanofibres The chiral configuration of the amorphous TiO 2 and the helical stacking of the TiO 2 nanocrystals endowed the materials with OA, which was unambiguously detected by diffused reflection circular dichroism (DRCD). 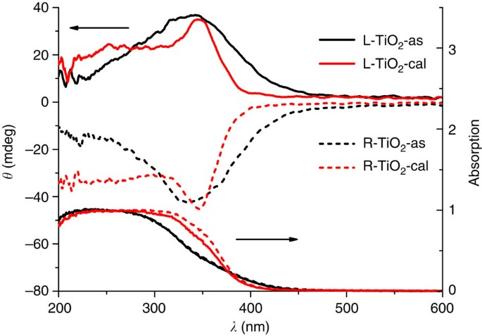Figure 4: Ultraviolet–vis and DRCD spectra of antipodal as-prepared and calcined chiral TiO2fibres. Ultraviolet–vis and DRCD spectra of antipodal as-prepared (L-TiO2-as and R-TiO2-as) and calcined (L-TiO2-cal and R-TiO2-cal, 550 °C) chiral TiO2fibres that show the ultraviolet absorption features and mirror-image CD signals that occurred at the TiO2semiconductor absorption band. Figure 4 shows the DRCD and ultraviolet–visible (ultraviolet–vis) spectra of two pairs of antipodal lipid–TiO 2 hybrid and calcined TiO 2 . The ultraviolet–vis spectra of the four samples each exhibited a broad absorption band in the range of 200–400 nm, which was attributed to the electronic transition from the valence band to the conduction band of the TiO 2 semiconductor. Compared with the crystalline anatase, the amorphous TiO 2 consisted of crystallites smaller than 50 Å in diameter with electronic properties that differed from those of the bulk materials [21] . The absorption of the as-prepared lipid–TiO 2 exhibited a slight hypsochromic shift compared with the calcined lipid–TiO 2 , which was most likely due to the quantum size effect of semiconductor crystallites [21] . The yellow-colour and the long-tail absorption at wavelengths greater than 400 nm were attributed to narrowing of the band gap in the electronic structure due to the presence of organics on the TiO 2 (ref. 22 ). The antipodal left- and right-handed amorphous TiO 2 showed strong mirror-image critical dimension (CD) signals with a peak at ~335 nm corresponding to the absorption edges, which indicates that the OA of the chiral TiO 2 was primarily a reflection of the intrinsic electronic structure. These samples selectively reflect left- or right-handed circularly polarized light in the ultraviolet absorption region through a vicinal effect of helically arranged TiO 2 species. As expected, a slight bathochromic shift was observed in the CD signals (~350 nm) for the calcined anatase samples in the corresponding absorption region, which indicates that the helical stacking of TiO 2 crystals that were in close proximity induced strong CD signals. On the basis of structural considerations, it can be considered that the dynamic Coulomb interaction under dissymmetric field electron transition from the valence band to the conduction band of TiO 2 results in its OA [23] , [24] . As known, the interaction between excited states of chromophores in chiral environments, called the exciton coupling, often give a split bisignate CD curves with the zero-crossing at the maximum absorption [25] , [26] . However, such exciton coupling spectra effect was not observed in the chiral TiO 2 material. The reason for it may be that inorganic such as metals and metal oxides always have a manifold of electronic transitions and, thus, the electronic transition-based circular dichroism may contain multiple absorption bands resulting in their overlaping [27] . Figure 4: Ultraviolet–vis and DRCD spectra of antipodal as-prepared and calcined chiral TiO 2 fibres. Ultraviolet–vis and DRCD spectra of antipodal as-prepared (L-TiO 2 -as and R-TiO 2 -as) and calcined (L-TiO 2 -cal and R-TiO 2 -cal, 550 °C) chiral TiO 2 fibres that show the ultraviolet absorption features and mirror-image CD signals that occurred at the TiO 2 semiconductor absorption band. Full size image Dual OA by induced chiral assembly Such long-range anisotropy of TiO 2 could be expected to direct the epitaxial self-assembly of the guest molecules. Porphyrins were selected as example, because they have aroused much popular interest for the inherent electronic and optical properties. 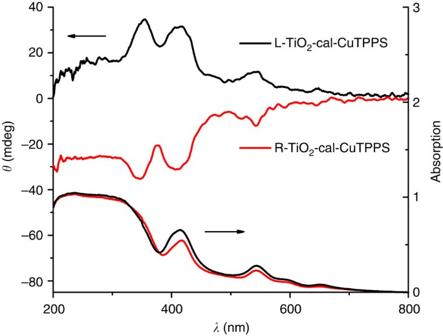Figure 5: Ultraviolet–vis and DRCD spectra of CuTPPS assembled on calcined chiral TiO2fibres. Ultraviolet–vis and DRCD spectra of CuTPPS assembled directly on the calcined (L-TiO2-cal and R-TiO2-cal, 550 °C) chiral TiO2fibres that show the ultraviolet absorption features and mirror-image CD signals of the chiral TiO2–CuTPPS complex. Figure 5 shows the DRCD and ultraviolet–vis spectra of copper (II) complexed tetra-4-sulfonatophenyl-porphyrin (CuTPPS) assembled on the chiral TiO 2 at pH=7.4. The ultraviolet–vis spectra of both complexes show a broad Soret band with 417 nm and four weak Q bands were well resolved in the region of 500–700 nm. However, no obvious blue or red shift of these bands was observed to support the existence of an H or J aggregate. It showed that the CuTPPS disks are almost monodispersed on the chiral TiO 2 with a weak coupling effect of the conjugated ring systems. Nevertheless, a pair of mirror-image DRCD spectra at the Soret and Q bands indicates that CuTPPS was helically stacked on the surface of TiO 2 mesocrystals due to helical arrangement of individual crystal of the chiral TiO 2 (ref. 28 ). Such a TiO 2 /CuTPPS complex is worth expecting to be used in dye-sensitized solar cells, photocatalysts, and so on, because that the unique arrangement of photosensitizer on semiconductor materials with the coupling effect could facilitated electron transfer and reduce recombination of the photogenerated electron-hole pairs arising from electronic interactions at their interface [29] , [30] , [31] . Figure 5: Ultraviolet–vis and DRCD spectra of CuTPPS assembled on calcined chiral TiO 2 fibres. Ultraviolet–vis and DRCD spectra of CuTPPS assembled directly on the calcined (L-TiO 2 -cal and R-TiO 2 -cal, 550 °C) chiral TiO 2 fibres that show the ultraviolet absorption features and mirror-image CD signals of the chiral TiO 2 –CuTPPS complex. Full size image To the best of our knowledge, this is the first synthesis of an inorganic material with OA that has attributed to the electronic transition, which differs from optically active inorganic materials in which the OA is induced from the scattering or refraction of light and metal plasmonic oscillations. ETOA materials exhibit OA in the wavelength region that depends on the inorganic materials and their self-electronic state; therefore, it is possible to control the wavelength of the OA in the full ultraviolet–vis region by using different inorganic compounds. Such chiral materials have a clear advantage over both chiral organic assemblies and chiral nanoparticles supported by organics due to their increased physical robustness, which yields a permanent molecular inorganic chiral property. Microscopic chirality in inorganic materials could present both daunting challenges and significant opportunities in various research areas, such as physics, chemistry, material science, bioscience, devices (for example, optical, electrical, and mechanical), and the origin of life. Preparation of optically active helical TiO 2 nanofibres The helical TiO 2 nanofibres can be synthesized over a wide range of molar compositions of C 18 - D -Glu:TDA:MeOH:H 2 O=1: x : y :55962, where x and y can be adjusted in the range of 5–60 and 3,800–6,600, respectively. A temperature of 45–60 °C is favourable for the formation of helical fibres. In a typical synthesis, C 18 - D -Glu (0.03 g, 0.08 mmol) was dissolved in a mixture of methanol (13.6 g) and deionized water (80 ml) while stirring at room temperature. After the mixture was stirred for 10 min, TDA (0.29 g, 75% in isopropanol, purchased from TCI) was added to the mixture with stirring at 55 °C. The mixture was allowed to react at 55 °C with stirring for 2 h. The products were collected by centrifugal separation and dried by freeze drying at −60 °C, which resulted in a pale yellow powder. All organics in this product were removed by calcination at 550 °C, and crystalline anatase was obtained. The method for the synthesis of the helical TiO 2 nanofibres using C 18 - L -Glu is the same as the above. Inducing self-assembly of CuTPPS on the chiral TiO 2 CuTPPS (5 mg, purchased from TCI) was dissolved in 5 ml of ion-exchanged water and a desired amount of aqueous NaOH solution (0.1 mmol l −1 ) with stirring for 2 min at room temperature. The calcined TiO 2 nanofibres (50 mg) were then dispersed in the above solution with stirring for 2 min, and then standing for 20 min at room temperature. The orange solid was separated with a centrifuge and dried by freeze drying at −60 °C. Characterization The morphology of the chiral TiO 2 nanofibres was observed with SEM (JEOL JSM-7401F) with an accelerating voltage of 1.0 kV. HRTEM images were taken with a JEOL JEM-2100 microscope operating at 200 kV. Powder X-ray diffraction patterns were recorded on a Rigaku X-ray diffractometer D/MAX–2200/PC equipped with Cu K α radiation (40 kV, 20 mA). Ultraviolet and DRUV spectra were taken by using a Shimadzu UV-2450 spectropolarimeter fitted with DRUV apparatus. CD and DRCD spectra were taken by using a JASCO J-815 spectropolarimeter fitted with DRCD apparatus. The N 2 adsorption/desorption isotherms were obtained at 77 K by using a Quantachrome NOVA 4200E surface area and pore-size analyser. Fourier transform infrared spectra were recorded on a Perkin-Elmer Paragon 1000 spectrometer with a resolution of 2 cm −1 using the KBr method. How to cite this article: Liu, S. et al. Synthesis of chiral TiO 2 nanofibre with electron transition-based optical activity. Nat. Commun. 3:1215 doi: 10.1038/ncomms2215 (2012).